Coiling and maturation of a high-performance fibre in hagfish slime gland thread cells The defensive slime of hagfishes contains thousands of intermediate filament protein threads that are manufactured within specialized gland thread cells. The material properties of these threads rival those of spider dragline silks, which makes them an ideal model for biomimetic efforts to produce sustainable protein materials, yet how the thread is produced and organized within the cell is not well understood. Here we show how changes in nuclear morphology, size and position can explain the three-dimensional pattern of thread coiling in gland thread cells, and how the ultrastructure of the thread changes as very young thread cells develop into large cells with fully mature coiled threads. Our model provides an explanation for the complex process of thread assembly and organization that has fascinated and perplexed biologists for over a century, and provides valuable insights for the quest to manufacture high-performance biomimetic protein materials. The hagfish gland thread cell (GTC) is remarkable because of the strength of the thread it produces [1] , but also because of the thread’s impressive length ( ∼ 150 mm) [2] , its exquisite packaging within the cytoplasm [3] , [4] , and its ability to deploy rapidly in seawater without tangling [5] . Although the exact site of thread assembly is unknown, it is most likely the region just apical to the nucleus where the thinnest regions of the thread are found [6] , [7] . As the GTC matures, loops of thread are generated and organized by an unknown mechanism into what have been referred to as conical loop arrangements [4] . The continuous coiling of the thread into these conical loop arrangements results in a ‘skein’ that is comprized of about 15–20 conical layers of thread loops [4] . In mature cells, these highly organized loops fill most of the cell volume. While others have attempted to describe how the thread is organized within thread cells [3] , [4] , [6] , these studies were limited by their reliance on surface imaging (scanning electron microscopy (SEM) and light microscopy) or snapshots of the skein interior from cross-sections (transmission electron microscopy (TEM)). Our goal was to understand the three-dimensional (3D) morphology of the coiled slime thread in both mature and immature GTCs in order to gain insight into possible mechanisms of thread production and coiling. The mature slime thread consists mainly of two intermediate filament (IF) proteins, α and γ [8] , [9] . Immature slime threads contain both 12-nm diameter IF and microtubules (MT), but it is unclear which of these elements appears first in nascent portions of the thread. Early in its development, the thread also appears to be wrapped with a distinctive ∼ 12-nm diameter filament [5] of unknown function. The most dramatic change in thread ultrastructure corresponds with the compaction of 12-nm diameter IFs into a dense superstructure in which discrete IFs are no longer visible and MT become surrounded by an electron lucent space presumably freed up by IF compaction [6] , [7] . This shift in thread ultrastructure likely corresponds with the post-translational modification of IF proteins within mature GTCs [8] , [9] ; it also coincides with the loss of the wrapping filament and the appearance of a fluffy rind around the thread periphery [6] , [7] . In fully mature threads, MTs are absent [6] , [7] , the spaces they occupy are completely filled in, the fluffy rind is gone, and adjacent threads conform to each other leaving only a narrow space of about 40 nm between them. In this study, we use light and electron microscopy as well as 3D imaging and modelling to describe the pattern of slime thread coiling within developing gland thread cells. Our results lead us to a new understanding of slime thread coiling and maturation, and confirm the observations made by other researchers in a different genus of hagfishes, suggesting that GTC and slime thread maturation may be highly conserved among the hagfishes. Morphology of developing GTCs We confirmed using light microscopy that GTCs originate in the slime gland epithelium and move towards the gland lumen as they mature [3] ( Fig. 1a ). SEM of isolated skeins that had cracked open revealed the morphology of conical loop arrangements at various places in the skein ( Fig. 1b ). To gain deeper insight into thread organization, morphology and maturation, we used TEM to observe GTCs at various stages in development ( Fig. 1c ). While changes to the length, diameter and morphology of the thread are the most obvious changes in the ultrastructure of maturing GTCs, changes in nuclear size and shape are also dramatic. The nucleus of an immature (that is, recently differentiated) GTC, identifiable because of its large prominent nucleolus, is round and occupies the majority of the cell volume. As the number of mitochondria and ribosomes in the GTC increase and thread synthesis begins, the nucleus becomes longer and more conical, eventually adopting a spindle shape with a flared base. In fully mature cells, the nuclear spindle recedes, leaving only a hemispherical nuclear cap outside the coiled skein. 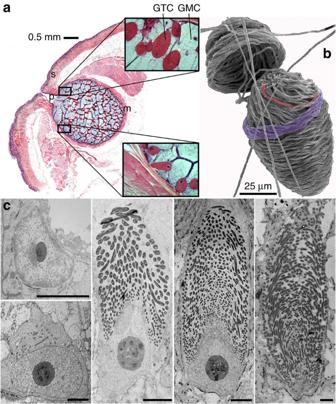Figure 1: Hagfish slime gland, gland thread cells and thread skeins. (a) H&E-stained cross-section of slime gland showing: gland thread cells (GTC), gland mucus cells (GMC), gland pore (p), striated muscle around gland (m) and skin (s). Insets show an immature GTC near the gland epithelium, and a mature GTC within the gland lumen. (b) SEM of coiled thread from a mature GTC that has broken open, revealing the organization of staggered loops (partially highlighted in red), which form layers of conical loop arrangements that spiral around the skein (one layer highlighted in purple). (c) Developmental progression ofM. glutinosaGTCs revealed with TEM illustrating dramatic changes in nuclear size and shape. Immature GTCs lacking a slime thread can be identified by their prominent nuclei and nucleoli. As the slime thread increases in length and diameter, the nucleus becomes more spindle-like, eventually receding to the basal end of the cell in mature cells. Scale bar, 5 μm. Figure 1: Hagfish slime gland, gland thread cells and thread skeins. ( a ) H&E-stained cross-section of slime gland showing: gland thread cells (GTC), gland mucus cells (GMC), gland pore (p), striated muscle around gland (m) and skin (s). Insets show an immature GTC near the gland epithelium, and a mature GTC within the gland lumen. ( b ) SEM of coiled thread from a mature GTC that has broken open, revealing the organization of staggered loops (partially highlighted in red), which form layers of conical loop arrangements that spiral around the skein (one layer highlighted in purple). ( c ) Developmental progression of M. glutinosa GTCs revealed with TEM illustrating dramatic changes in nuclear size and shape. Immature GTCs lacking a slime thread can be identified by their prominent nuclei and nucleoli. As the slime thread increases in length and diameter, the nucleus becomes more spindle-like, eventually receding to the basal end of the cell in mature cells. Scale bar, 5 μm. Full size image 3D structure of the coiled slime thread To understand the precise patterning of staggered loops, we used focused ion beam scanning electron microscopy (FIB-SEM) to generate a 3D model of thread coiling ( Fig. 2a ) ( Supplementary Movie 1 ). By tracing the 3D structure of a dozen continuous loops using Mimics (v. 15.01) software, we were able to elucidate for the first time the morphology of thread loops within an immature GTC; this enabled us to define the precise spatial relationship between adjacent loops ( Fig. 2b ) ( Supplementary Movie 2 ). With these data we constructed a 3D model using Maya 2013 software of thread coiling that is built around a repeating loop structure ( Fig. 2c ) ( Supplementary Movie 3 ). This model reproduces many of the most salient features of natural thread skeins, specifically, the spiralling nature of the conical loop structures, the nesting of these structures within each other, as well as the cabled appearance of the skein where the thread runs circumferentially along the skein surface. 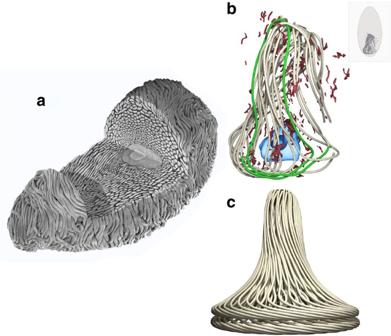Figure 2: 3D reconstruction of thread coiling within an immature GTC from the FIB-SEM data. (a) Stacks of images from FIB-SEM were assembled into a 3D volume using Mimics software. This image was created by combining axial and transverse sections of the rendered volume with an SEM image of a separate complete thread skein. (b) Segmentation of a dozen continuous loops within a developing GTC revealed the precise 3D pattern of thread coiling (single loop in green). 3D reconstruction of the nucleus (light blue), nucleolus (dark blue) and mitochondria (maroon) shows the relative position of these structures to the developing thread. The loops shown are not the most recent ones laid down on the nucleus (these were too small to follow), but they do reflect nuclear shape at the time of synthesis. Inset shows the position of the rendered structures within the cell. (c) Based on the 3D structure of a single loop and its relationship to adjacent loops, our model (built in Maya 2013) reproduces the spiralling nature of the conical loops, the nesting of these conical structures, as well as the cabled appearance of the skein where the thread runs circumferentially along the skein surface. Figure 2: 3D reconstruction of thread coiling within an immature GTC from the FIB-SEM data. ( a ) Stacks of images from FIB-SEM were assembled into a 3D volume using Mimics software. This image was created by combining axial and transverse sections of the rendered volume with an SEM image of a separate complete thread skein. ( b ) Segmentation of a dozen continuous loops within a developing GTC revealed the precise 3D pattern of thread coiling (single loop in green). 3D reconstruction of the nucleus (light blue), nucleolus (dark blue) and mitochondria (maroon) shows the relative position of these structures to the developing thread. The loops shown are not the most recent ones laid down on the nucleus (these were too small to follow), but they do reflect nuclear shape at the time of synthesis. Inset shows the position of the rendered structures within the cell. ( c ) Based on the 3D structure of a single loop and its relationship to adjacent loops, our model (built in Maya 2013) reproduces the spiralling nature of the conical loops, the nesting of these conical structures, as well as the cabled appearance of the skein where the thread runs circumferentially along the skein surface. Full size image Changes in thread ultrastructure with cell maturation Our TEM studies largely substantiate observations of thread development described in other species of hagfishes [6] , [7] , [9] , but they also add to our understanding of the ultrastructural changes that take place during thread maturation ( Fig. 3a,b ). Our results clearly establish that thread production starts with a small bundle of IFs in a paranuclear region rich in mitochondria and ribosomes. The thread increases in both length and width via the addition of IFs and eventually via the incorporation of MTs. The youngest threads are only 2–3 IFs in diameter (about 30 nm) and more mature ones are about 30 IFs in diameter (about 400 nm). The wrapping filament is clearly visible in immature threads, but it is not clear whether the filament spirals around the thread at a steep angle [6] or exists as separate rings ( Fig. 3c ). The condensation of IFs corresponds not only with the loss of the wrapping filaments, but also with the appearance of the fluffy rind that has been described by others [6] , [7] . High power TEM revealed the presence of MTs within the post-IF condensation thread ( Fig. 3a,d ), as described by others [6] , [7] , as well as evidence that the MTs penetrate the thread from the side ( Fig. 3d ). 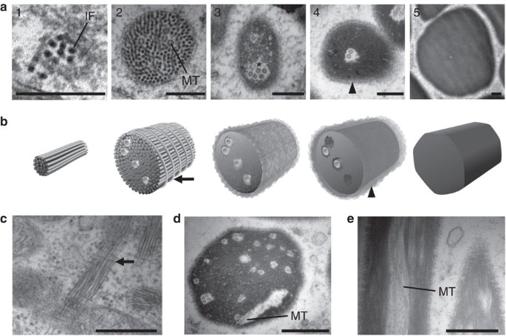Figure 3: Developmental series of thread ultrastructure. (a) TEM sections of slime threads from very immature to fully mature GTCs. The thread depicted in (1) consists of a bundle of about ten, 12-nm IFs. Threads increase in girth by the addition of more IFs, and eventually by the addition of MTs (2). In the next stage (3), 12-nm IFs become more tightly packed, which creates electron lucent halos (asterisk) around the MTs. Further IF compaction is accompanied by the appearance of a fluffy rind (arrowheads) on the thread surface (4), which likely corresponds to the direct addition of IF subunits or proteins to the thread rather than the bundling of mature IFs. In the final stage, IF proteins compact further, MTs are lost, the spaces they occupied are filled in, and the fluffy rind disappears. In fully mature GTCs, the thread takes up the vast majority of the cell volume and adjacent threads are packed so tightly that they conform to each other (5). Scale bars are all 200 nm. (b) Models of thread development corresponding to each of the stages depicted in (a). The second panel illustrates the 12-nm diameter filament (arrows) that wraps around the thread at this stage in development (c) Young thread from stage (2) showing the wrapping filament (arrow), which is evident as regularly spaced circular sections and corresponding lines that cross the thread at an average angle of about 86°. (d) Cross-section of a thread from stage (4) showing a MT penetrating from the side (3). (e) TEM of thread longitudinal section depicting MTs within a developing thread. Scale bars, 500 nm (c–e). Figure 3: Developmental series of thread ultrastructure. ( a ) TEM sections of slime threads from very immature to fully mature GTCs. The thread depicted in (1) consists of a bundle of about ten, 12-nm IFs. Threads increase in girth by the addition of more IFs, and eventually by the addition of MTs (2). In the next stage (3), 12-nm IFs become more tightly packed, which creates electron lucent halos (asterisk) around the MTs. Further IF compaction is accompanied by the appearance of a fluffy rind (arrowheads) on the thread surface (4), which likely corresponds to the direct addition of IF subunits or proteins to the thread rather than the bundling of mature IFs. In the final stage, IF proteins compact further, MTs are lost, the spaces they occupied are filled in, and the fluffy rind disappears. In fully mature GTCs, the thread takes up the vast majority of the cell volume and adjacent threads are packed so tightly that they conform to each other (5). Scale bars are all 200 nm. ( b ) Models of thread development corresponding to each of the stages depicted in ( a ). The second panel illustrates the 12-nm diameter filament (arrows) that wraps around the thread at this stage in development ( c ) Young thread from stage (2) showing the wrapping filament (arrow), which is evident as regularly spaced circular sections and corresponding lines that cross the thread at an average angle of about 86°. ( d ) Cross-section of a thread from stage (4) showing a MT penetrating from the side (3). ( e ) TEM of thread longitudinal section depicting MTs within a developing thread. Scale bars, 500 nm ( c – e ). Full size image The changes in nuclear shape observed using TEM correspond with changes in the morphology of the conical loop arrangements observed using FIB-SEM, and suggest that the nucleus acts as a template on which the staggered loops form. Specifically, the loops making up the cones are short near the apical tip of the cell when the cell nucleus is round, and considerably longer towards the basal end as the nucleus becomes more spindle shaped. In this way, the nucleus likely provides an obstruction that limits where the thread can be deposited as it elongates from its site of synthesis. Our data and model suggest that the ascending and descending portions of the conical loops are directly shaped by the nucleus, whereas the circumferential runs, which form the base of each conical loop, are laid down in the basal groove where the nucleus and plasma membrane converge ( Fig. 1c ). In nearly mature GTCs, the nucleus is reduced to only a fraction of its former size, and its full retreat in a basal direction leads to very short circumferential runs and loops consisting of mostly back and forth axial runs, called ‘inner core loops’ by Fernholm [4] ( Fig. 4 ). While our model explains many aspects of slime thread morphology, it does not explain how the precise staggering of loops arises. The fact that each successive loop is translocated in a clockwise direction relative to its younger neighbouring loop is suggestive of a wheel-like mechanism at work. Although wheels are extremely rare in biology [10] , thread coiling may involve just such a mechanism. 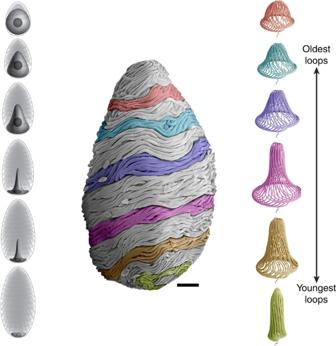Figure 4: Temporal and spatial models of thread assembly and coiling in GTCs. GTC growth and maturation is characterized by dramatic changes in nuclear size and morphology (left), which correspond with the shape of conical loop arrangements laid down during successive stages of thread production (right). Regular staggered loops are laid down in the space defined by previous loops and the apical surface of the nucleus, and their morphology changes as the nucleus becomes more spindle shaped and retreats towards the basal end of the cell. The result of manufacturing the skein in the manner depicted is a mature, ovoid skein that can be ejected through the gland pore and unravel to its full extended length of∼150 mm without tangling. Scale bar, 10 μm. Figure 4: Temporal and spatial models of thread assembly and coiling in GTCs. GTC growth and maturation is characterized by dramatic changes in nuclear size and morphology (left), which correspond with the shape of conical loop arrangements laid down during successive stages of thread production (right). Regular staggered loops are laid down in the space defined by previous loops and the apical surface of the nucleus, and their morphology changes as the nucleus becomes more spindle shaped and retreats towards the basal end of the cell. The result of manufacturing the skein in the manner depicted is a mature, ovoid skein that can be ejected through the gland pore and unravel to its full extended length of ∼ 150 mm without tangling. Scale bar, 10 μm. Full size image Interactions between the IFs known as nuclear lamins and the inner nuclear membrane are well described [11] , [12] , but less is known about how the outer nuclear membrane interacts with cytoplasmic elements [13] , [14] . The patterning of slime thread coiling by the GTC nucleus may provide a new model for exploring these interactions in detail. Our data also raise questions about how such dramatic changes in nuclear size and shape are regulated. Our observations are consistent with the hypothesis that elongation occurs at a single site near the apical tip of the nucleus [6] , but the mechanism of elongation remains elusive. The role of intra-thread MTs is also unclear, although they may be involved in the delivery of IFs and/or IF subunits [15] , [16] to the interior of the growing thread. Indeed, TEM and FIB-SEM images both demonstrate MTs within the thread and penetrating the thread from the side ( Fig. 3d ). The 12-nm filament that wraps around the thread ( Fig. 3b,c ) before the IFs condense is also puzzling. Downing et al. [6] propose that the filament is involved in the addition of IF to the growing thread, but how exactly this would work is difficult to imagine. We suggest that the wrapping filaments may prevent the merging of adjacent loops, which would have obvious negative effects on thread deployment and ultimately on the function of the slime [1] . Two other cell types, the hagfish epidermal thread cell and the lamprey skein cell, notably also produce thick helical IF bundles [17] , [18] , in contrast to the branching networks of IFs that are far more common in metazoan cells [19] . In hagfish GTCs, this ability to produce a single, unbranched IF bundle has been taken to the extreme and may be one of the key adaptations that allowed hagfishes to evolve their remarkable fibrous defensive slime. Our results confirm that the condensation of discrete 12-nm IFs is an important step in slime thread maturation and occurs in all the species of hagfish examined thus far [6] , [7] . Previous work suggests that IF condensation may be regulated by phosphorylation of γ [8] , [9] , which may also mark a transition to thread growth mediated by the direct addition of IF proteins to the condensed thread rather than the addition of discrete IFs to a growing bundle. Recent efforts to make fibres from solubilized hagfish slime thread proteins and the IF protein vimentin yielded threads with promising material properties, but they were clearly inferior to native slime threads [20] , [21] . The changes in thread ultrastructure documented here suggest that the outstanding mechanics of native slime threads likely arise via careful control of protein structure from IF subunits to mature IFs to dense IF superstructure. Unravelling the biochemical and biophysical mechanisms underlying these transitions may lead us to new methodologies for the production of sustainable high-performance protein materials. Animal collection, care and procedures Specimens of Atlantic hagfish ( Myxine glutinosa ) (used for TEM and FIB-SEM) were collected in Passamaquoddy Bay, New Brunswick, Canada. Pacific hagfish ( Eptatretus stoutii ) (used for gland histology and whole skein SEM) were obtained from the Bamfield Marine Station, Bamfield, BC, Canada. Hagfishes were housed at the Hagen Aqualab at the University of Guelph in 2000-L, environmentally-controlled, aquatic recirculation units containing artificial seawater (10 °C, 34%). Hagfish were anaesthetized using a clove-oil anaesthetic protocol [5] . Following anaesthesia the slime glands of the hagfish were electrostimulated (60 Hz, 18 V) using a Grass SD9 electric stimulator (Grass Instruments, Quincy, MA, USA). For harvested glands, electrostimulation was performed 1 or 2 weeks before tissue collection to increase the ratio of immature: mature cells [9] . Hagfish were killed by severing the notochord and dorsal nerve cord directly posterior to the cranium with a large scalpel. All housing and feeding conditions were in accordance with the University of Guelph Animal Use Protocol 09R128. SEM of thread skeins from slime exudates Slime exudate was collected from anaesthetized hagfish as described above and stabilized in an aqueous stabilization buffer (0.9 M sodium citrate, 0.1 M PIPES, pH 6.7). Thread skeins were separated from much smaller mucin vesicles by filtering through 53 μm Nylon mesh. Skeins were fixed in 3% paraformaldehyde in phosphate-buffered saline (PBS) and transferred into 30% ethanol and dehydrated using the following ethanol series for 15 min each: 30, 50, 70, 95 and 100% (3 × ). The same dehydration series was used for tissues prepared for TEM and histology (see below). Dehydrated skeins were critical point dried and then sputter coated using an Emitech K550 Sputter Coater (Emitech Ltd, Ashford, Kent, England) to produce an ∼ 12-nm Au/Pd coating (20 mA for 2 min). The prepared skein samples were then observed using a Hitachi S-570—Scanning Electron Microscope (Hitachi High Technologies, Tokyo, Japan) and images were captured using the Quartz PCI—Image Management System, v. 8.5. Slime gland fixation and embedding Killed hagfish were dissected by first making a 6-cm incision down the dorsal midline starting from the rostral end. Perpendicular cuts from this incision to the ventral midline created a rectangular flap of skin on each side. By carefully pulling the flap ventrally and away from the muscle tissue, the slime glands attached to the skin at the gland pore were pulled from between the large myotomal bands of skeletal muscle running dorso-ventrally along the length of the hagfish. Fine forceps were used to grasp the capsule of each exposed gland, and to gently pull it away from the skin to expose the gland pore. Iridectomy scissors were used to cut the slime gland pore where it attached to the epidermis. Following excision, the slime glands were transferred into a culture dish containing buffered fixative. For TEM and SEM, a fixative solution containing 3% paraformaldehyde and 3% glutaraldehyde in 0.1-M sodium cacodylate was used, followed by 3–10 min rinses with cacodylate buffer. Following fixation, glands were post-fixed with osmium tetroxide (1% in 0.1-M sodium cacodylate) and en bloc stained in a 2% uranyl acetate in 0.1-M sodium cacodylate solution. Fixed, osmicated, stained and dehydrated glands were plastic embedded for TEM and FIB-SEM using a Polysciences Poly/Bed812 (Luft formulations) embedding kit (Polysciences Inc. Warrington, PA). For histology, glands were fixed in 3% paraformaldehyde in PBS and rinsed three times for ten minutes in PBS and dehydrated using the ethanol series described above. Fixed and dehydrated slime glands were paraffin embedded at the University of Guelph Animal Health Laboratory using standard protocols. Hagfish tissues were sectioned using a microtome to 4 μm sections and mounted on glass slides for staining with hematoxylin and eosin (H&E). FIB-SEM Before mounting, plastic-embedded glands were sectioned to expose the cells at the periphery and in the lumen of the gland. This was performed using a Porter-Blum MT-1 manually-driven ultramicrotome (Ivan Sorvall, Inc.). Samples were sputter coated with a 5-nm gold coating (Model S150B; Edwards; England) and mounted for FIB-SEM on aluminium pin stubs (12.7 mm diameter) using silver paint. Embedded GTCs were milled away in 90 nm sections using a gallium-focused ion beam (FIB image probe 30 kV:80 pA, EHT=5 kV) and SEM images were collected after each layer was ablated. 3D model of continuous thread loops from FIB-SEM data Grayscale image stacks obtained from FIB-SEM experiments were imported into a 3D visualization software package (Mimics v. 15.01, Materialise NV, Leuven, Belgium) and a length of thread was segmented by manually masking its cross-section over the course of about a dozen staggered loops. Nucleus, nucleolus and mitochondria were individually segmented and rendered as separate 3D objects. 3D objects were exported from Mimics into Maya 3D animation software (v. 2013, Autodesk Inc. San Rafael, CA, USA) for further editing and the production of a high-resolution colour image and movie. Brightfield imaging H&E-stained hagfish tissue slides were visualized using a Nikon Eclipse 90i microscope. Brightfield colour images were taken using a Q-imaging E Xi 12-bit colour camera (Q-Imaging; Surrey, British Columbia, Canada) driven by NIS Elements AR software. TEM TEM was performed at the University of Guelph’s Electron Microscopy Unit using a Philips CM10 (tungsten filament 80 kV) outfitted with a top mount SIS/Olympus Morada 11MP CCD camera. Sections were cut between 20 and 60 nm using a Porter-Blum MT-1 manually-driven ultramicrotome and stained with uranyl acetate (2%) and lead citrate (1%) following sectioning. 3D modelling of skein coiling and organization A 3D model of thread coiling was created using Maya 2013 software starting with a single segmented thread loop imported from Mimics. By replicating the single loop and joining it end to end, we created a model of two complete conical loop arrangements. The repeating loop was given a circumferential run of 60 degrees, and each loop was offset by its neighbour above it by a distance of one fifth of a thread diameter in the axial dimension. Use of these parameters resulted in conical loop arrangements that best approximated the most salient features of natural skeins. How to cite this article: Winegard, T. et al. Coiling and maturation of a high performance fibre in hagfish slime gland thread cells. Nat. Commun. 5:3534 doi: 10.1038/ncomms4534 (2014).